A mutation burst during the acute phase ofHelicobacter pyloriinfection in humans and rhesus macaques The evolution rate and genetic changes that occur during chronic infection with Helicobacter pylori have been analysed, but little is known about the genomic changes during the initial, acute bacterial infection phase. Here we analyse the rate and pattern of genome evolution in H. pylori from the genomes of two input strains isolated from human volunteers with asymptomatic infection, and the genomes of two output strains collected 20 and 44 days after re-infection. Similarly, we analyse genome evolution in bacteria from the genome sequences of input and output strains sequentially taken after experimental infection of a rhesus macaque. The estimated mutation rate reveals a mutation burst during the acute infection phase that is over 10 times faster than the mutation rate during chronic infection, and orders of magnitude faster than mutation rates in any other bacteria. The elevated frequency of mutations in outer membrane protein genes suggests that the mutation burst facilitates rapid host adaptation of the bacteria. The stomach bacterium Helicobacter pylori has infected anatomically modern humans since their origins [1] , [2] , which implies perfect adaptation of the bacterial parasite to its human host. This remarkable adaptive capacity can be partly attributed to the enormous plasticity of the Helicobacter genome [3] caused by high mutation and recombination rates [4] , [5] , [6] , and by the ability for aberrant genomic rearrangements and incorporation of non-homologous DNA. This results in an exceptionally high sequence diversity among strains that were isolated from unrelated human hosts [1] , [2] , [7] , [8] , and in an H. pylori core genome that consists of only ~1,100 genes while the other ~400–500 genes per strain are strain-specific and variably present [9] . The initial infection with H. pylori induces an acute polymorphonuclear (PMN) reaction, most likely owing to the activation of the innate immune system. The acute inflammatory response involves the release of reactive oxygen and nitrogen species that were shown to trigger mutations and intra-chromosomal recombination in vitro [10] . After 2–4 weeks, the acute inflammation subsides and develops into a less severe chronic active gastritis, characterized by infiltration with PMNs, Th1-biased CD4+ T cells, plasma cells and even dendritic cells, which generally persists throughout the host’s life. Numerous genomic changes have been identified in studies where sequential H. pylori isolates have been recovered several years apart from patients with chronic infection. Whole-genome microarray analyses identified gene acquisitions and gene losses [11] . In addition, sequencing of gene fragments [4] , [12] , [13] and whole-draft genomes [5] , [6] revealed point mutations, imported DNA fragments and extensive recombination with co-colonizing strains, whereby genes encoding outer membrane proteins (OMPs) were at significantly increased frequency among the imported DNA fragments, suggesting diversifying selection [5] . During chronic infection, sequence differences accumulated in a clock-like manner [4] at a median mutation rate of 1.55 × 10 −5 changes per site per year and a recombination rate of 5.5 × 10 −5 per initiation site per year [5] , [6] . However, little is known about the mutation rate and genomic changes induced by the inflammatory response during the initial, acute bacterial infection. We hypothesized that the selection pressure during the acute inflammation would likely be higher than during chronic infection and result in a faster substitution rate. Here we test this hypothesis using experimental infection of human volunteers and a rhesus macaque. We determine the sequence differences that accumulate in the genomes of H. pylori output strains taken at several time points post infection, covering both the acute and chronic infection phases. Our genome comparisons reveal a mutation burst during the acute phase of H. pylori infection that is over 10 times faster than the mutation rate during chronic infection and orders of magnitude faster than mutation rates in any other bacteria. We show that genetic changes in OMP genes accumulate at elevated frequencies, suggesting that the mutation burst facilitates rapid adaptation of H. pylori to the individual human host. Re-infection of human volunteers Two human volunteers with asymptomatic H. pylori infections underwent gastroendoscopy and were then cured by antibiotic therapy. Eradication was confirmed 1 and 2 months later by two consecutive, clearly negative carbon-14 urea breath tests (UBTs). Three months later, the volunteers were re-infected with their own original strains BM012A and BM013A. H. pylori was grown from antral biopsy material that was collected during the initial endoscopic examinations as well as 20 days (strain BM013B) and 44 days (BM012B) after the re-infections. Visual inspection during the endoscopy as well as the histological analysis of the biopsies revealed moderate inflammation of the stomach epithelium ( Supplementary Fig. 1 ). Ultimately, H. pylori was eradicated with antibiotic treatment. We sequenced the genomes of the two re-infection input strains BM012A and BM013A, and of the two output strains BM012B and BM013B using a Roche 454-Titanium FLX sequencer to >60 × coverage, assembled the reads and closed the genomes by PCR and Sanger sequencing. The original strain BM012A that was used for the re-infection experiment possessed a genome with a length of 1,660,425 bp ( Fig. 1 ) that contained the cag pathogenicity island ( cag PAI), nine copies of the insertion element IS607 and an apparently non-functional vacA gene that was disrupted by a frameshift. Strain BM013A had a genome of 1,604,233 bp length that did not possess the cag PAI, and contained an apparently non-cytotoxic vacA allele (s2m2) and four IS607 copies. An additional IS607 copy was located on a 16.7-kb plasmid. 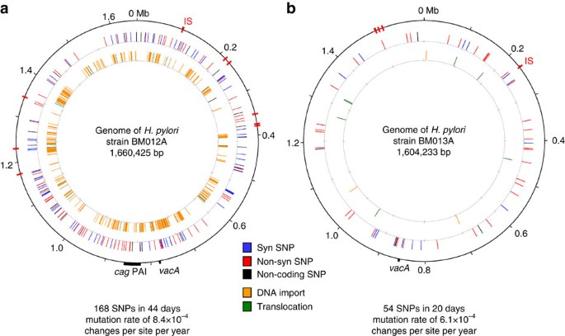Figure 1: Accumulation of SNPs and CNPs in theH. pylorigenomes after re-infection of human hosts. (Circle contents from outside to inside). Circle 1: Genomes ofH. pyloristrains BM012A (a) and BM013A (b) with the positions of IS607 (red), thecagPAI, thevacAgene and ticks every 100 kb. Circle 2: Distribution of non-coding (black), non-synonymous (red) and synonymous (blue) SNPs in the genomes of the output strains BM012B (168 SNPs) and BM013B (54 SNPs). Circle 3: Distribution of imported (orange) and translocated (green) DNA fragments in the genomes of the two output strains. syn SNP, synonymous SNP; non-syn SNP, non-synonymous SNP. Figure 1: Accumulation of SNPs and CNPs in the H. pylori genomes after re-infection of human hosts. (Circle contents from outside to inside). Circle 1: Genomes of H. pylori strains BM012A ( a ) and BM013A ( b ) with the positions of IS607 (red), the cag PAI, the vacA gene and ticks every 100 kb. Circle 2: Distribution of non-coding (black), non-synonymous (red) and synonymous (blue) SNPs in the genomes of the output strains BM012B (168 SNPs) and BM013B (54 SNPs). Circle 3: Distribution of imported (orange) and translocated (green) DNA fragments in the genomes of the two output strains. syn SNP, synonymous SNP; non-syn SNP, non-synonymous SNP. Full size image Changes in H. pylori genomes during human re-infection In comparison with the genome of the original strain BM012A, we identified 168 single-nucleotide polymorphisms (SNPs; separated from the next sequence difference by >200 bp of identical sequence on both sides [5] ) in the genome of the output strain BM012B that were scattered around the chromosome ( Fig. 1 , Table 1 , and Supplementary Tables 1 and 2 ). Variations in the length of homopolymeric nucleotide tracts were not included in the analysis. Twenty-two SNPs were located in non-coding regions, and 146 SNPs affected the coding regions of genes resulting in 73 synonymous and 73 non-synonymous mutations. In addition to SNPs, we identified 255 clusters of nucleotide polymorphisms (CNPs), which we defined as two or more sequence differences separated by <200 bp and flanked by >200 bp of identical sequence on both sides, similar to Kennemann et al . [5] Twenty-one CNPs likely originated from intra-chromosomal translocations, whereas 234 CNPs presumably resulted from imported foreign DNA ( Fig. 1 , and Supplementary Tables 1 and 3 ). The incorporated DNA fragments had a mean length of 740 bp (range 9–6, 192 bp), adding up to a total length of 173 kb, and likely resulted from 102 DNA fragments (groups of import) taken up from the environment. Table 1 SNPs in the genomes of the output strains BM012B and BM013B. Full size table The genome of strain BM013B contained 54 SNPs ( Fig. 1b , Table 1 , and Supplementary Tables 1 and 4 ), four of which were non-coding, whereas 50 were located in gene coding sequences and resulted in 15 synonymous and 35 non-synonymous mutations. In addition, we identified 10 CNPs, only three of which originated from import of foreign DNA, whereas the remaining seven CNPs likely arose by intra-chromosomal recombination ( Supplementary Tables 1 and 5 ). All nucleotide changes were located on the bacterial chromosome, whereas no polymorphisms were detected in the plasmid sequence. A mutation burst during the acute H. pylori infection phase Based on the 54 SNPs that had accumulated in the genome of strain BM013B within 20 days and 168 SNPs that had accumulated in the genome of strain BM012B within 44 days after re-infection, we calculated a total mutation rate of 6.1–8.4 × 10 −4 changes per site per year ( Fig. 1 and Supplementary Table 1 ) for H. pylori during the acute infection phase. This mutation rate was 40–50 times faster than the median mutation rate of 1.55 × 10 −5 (range 0.5–6.5 × 10 −5 ) that was estimated from whole genomes from paired sequential isolates during chronic infection [5] , [6] ( Supplementary Table 6 ), and orders of magnitude faster than mutation rates in other bacteria ( Supplementary Table 7 ). In addition, the mutation rate estimate from chronic infection likely represents an overestimation because of functional inactivation of mutation repair genes mutY and uvrC by frameshift mutations in the strain with the highest mutation rate ( Supplementary Table 6 ). Our data suggest different mutation rates during particular stages of an H. pylori infection, which we attempted to analyse in more detail. Since there were no additional H. pylori isolates from acute human infection available to us, we used experimental inoculation of a rhesus monkey that results in persistent infection and a histological gastritis similar to that seen in humans [14] , [15] . Previously, rhesus macaques were inoculated with the macaque adapted H. pylori strain J166 that contained a s1m1 vacA allele and a functional cag PAI that consisted of two fragments, cag1 through cagB and cagA , separated by 12.5 kb of sequence ( Supplementary Fig. 2 ). Biopsies were taken under anaesthesia after an overnight fast 1 week and 1, 2 and 6 months post-orogastric H. pylori infection [16] . We sequenced the genome of strain J166 (1,650,561 bp) on a Roche 454-Titanium FLX sequencer, and the genomes of 12 J166 macaque output (J166 output ) strains, three individual bacterial strains cultivated from each of the four biopsies on an Illumina MiSeq to an average coverage of × 200. 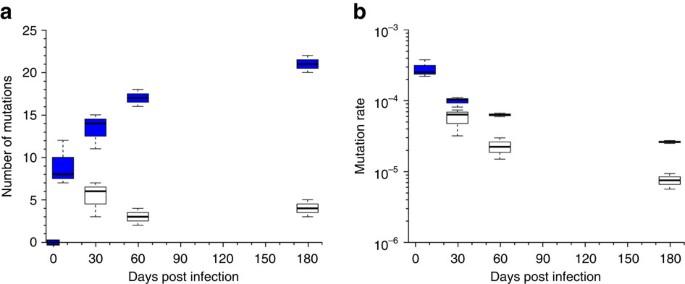Figure 2: Accumulation of SNPs and mutation rates in the macaque J166outputstrains. (a) Box-and-whisker plot of the cumulative number of mutations in three J166outputstrains each that were taken 1 week and 1, 2 and 6 months post infection (blue boxes). The adjusted number of mutations that accumulated in addition to the median number of mutations at the previous sampling point is shown in white boxes. (b) Box-and-whisker plot of the estimated mutation rate between the inoculation day and the sampling point (blue boxes). The estimated mutation rates between the inoculation and 1 week, between 1 week and 1 month, between 1 and 2 months, and between 2 and 6 months are shown as white boxes. The band inside the box represents the median, and the bottom and the top of the box are the first and the third quartiles, respectively. The whiskers indicate the range of the data. The number of point mutations in the J166 output strains increased in a time-dependent manner, but this increase was not linear: a median of 8 SNPs accumulated within 1 week post infection, a median of 14 SNPs within 1 month, 17 SNPs within 2 months and 21 SNPs within 6 months post infection ( Table 2 , Fig. 2a and Supplementary Fig. 2 ). The median number of mutations per sampling time corresponded to mutation rates of 2.5 × 10 −4 changes per site per year within 1 week, of 1.0 × 10 −4 within 1 month, of 6.3 × 10 −5 within 2 months and of 2.6 × 10 −5 within 6 months post inoculation ( Table 2 and Fig. 2b ), revealing a peak in the mutation rate at the beginning of the infection. The mutation burst of 2.2 × 10 −4 to 3.8 × 10 −4 within 1 week was close to the estimated mutation rate of 6.1–8.4 × 10 −4 during the re-infection of the human volunteers ( Fig. 1 ). The peak in the mutation rate was more prominent when the mutation rate was adjusted for the number of mutations that accumulated between the sampling points. On top of the eight SNPs that accumulated between the inoculation and sampling point on day 7, the median number of SNPs consecutively increased by six, three and four additional SNPs at the sampling points after 1, 2 and 6 months, respectively ( Fig. 2a and Table 2 ). This corresponded to median mutation rates of 2.5 × 10 −4 between the inoculation and 1 week, of 6.3 × 10 −5 between 1 week and 1 month, of 2.2 × 10 −5 between 1 and 2 months, and of 0.74 × 10 −5 between 2 and 6 months, emphasizing the mutation burst during the acute infection phase. The mutation rates of 2.2 × 10 −5 between 1 and 2 months and of 0.74 × 10 −5 between 2 and 6 months were within the range of those determined during chronic infection, indicating that the acute infection had likely subsided and changed into the chronic infection phase. Table 2 Number of accumulated SNPs and mutation rates in the J166 output strains. Full size table Figure 2: Accumulation of SNPs and mutation rates in the macaque J166 output strains. ( a ) Box-and-whisker plot of the cumulative number of mutations in three J166 output strains each that were taken 1 week and 1, 2 and 6 months post infection (blue boxes). The adjusted number of mutations that accumulated in addition to the median number of mutations at the previous sampling point is shown in white boxes. ( b ) Box-and-whisker plot of the estimated mutation rate between the inoculation day and the sampling point (blue boxes). The estimated mutation rates between the inoculation and 1 week, between 1 week and 1 month, between 1 and 2 months, and between 2 and 6 months are shown as white boxes. The band inside the box represents the median, and the bottom and the top of the box are the first and the third quartiles, respectively. The whiskers indicate the range of the data. Full size image Diversifying selection in H. pylori during host adaptation The 65 OMP encoding genes in the output strain BM012B contained 16 SNPs ( Table 1 ), which was significantly more than expected given the total of 146 SNPs in 1,591 coding genes (Fisher’s exact test, P =0.001914). Likewise, nine out of 73 non-synonymous SNPs ( Table 1 ) were located in OMP genes ( P =0.006657). 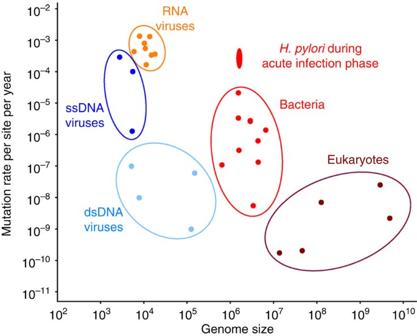Figure 3: Mutation rate versus genome size for bacteria and other biological entities. The estimatedH. pylorimutation rate during the acute infection phase was orders of magnitude faster than the mutation rate in other bacteria, comparable to the evolutionary rate of RNA viruses. Data points were taken from references inSupplementary Table 7. dsDNA, double-stranded DNA; ssDNA, single-stranded DNA. In addition, 26 out of the 302 genes (8.6%) that were affected by the 234 CNPs in strain BM012B that arose from recombination of imported DNA ( Supplementary Table 3 ) encoded OMPs, significantly more than the overall ratio of OMP genes in the genome (65/1,591 genes, 4.1%; P =0.003398). Similarly, two out of the six CNPs that affected genes in strain BM013B ( Supplementary Table 5 ) altered OMP encoding genes ( P =0.03823), namely hopM (intra-chromosomal translocation from hopF ) and hopZ (DNA import). OMP genes were also changed at high frequency in the rhesus macaque output strains, particularly the BabA adhesin encoding gene hopS that was altered in 11 of the 12 J166 output strains, indicating selection against this OMP ( Supplementary Tables 8–19 ). In addition, frameshift mutations in the essential cag PAI genes cagX and cagY in J166 output strains isolated after 2 and 6 months apparently abolished the function of the cag PAI type IV secretion system that delivers the immunogenic effector protein CagA into the epithelial cells, suggesting selection against a functional cag PAI ( Supplementary Fig. 2 and Supplementary Tables 14–19 ). The mutation burst of 2.2 × 10 −4 –8.4 × 10 −4 changes per site per year that we estimated for the acute H. pylori infection phase was over one order of magnitude faster than the H. pylori mutation rate of 0.91 × 10 −5 –1.85 × 10 −5 changes per site per year that was based on SNPs in 786 core genes in 40 H. pylori genome pairs [6] , and the median estimate of 1.55 × 10 −5 (range 0.5 × 10 −5 –6.5 × 10 −5 ) determined from sequential isolates obtained from patients with chronic infection [5] . This extraordinarily fast mutation rate during the acute infection phase is the highest mutation estimate so far for any bacteria, exceeding the substitution rate in other bacterial species by at least two orders of magnitude ( Fig. 3 and Supplementary Table 7 ). However, whole-genome data on bacterial changes during the initial infection phase, such as presented here for H. pylori , are missing for other (pathogenic) bacteria; most of the previous mutation rates were determined from sequential isolates obtained from chronic infection or were estimated from phylogenetic comparisons of bacterial lineages obtained over many years or decades. For example, the accumulated mutations in an Escherichia coli clone that persisted in a family for 3 years gave a rate of 2.26 × 10 −7 changes per site per year [17] . The genomic changes during chronic Pseudomonas aeruginosa infection in the airways of a cystic fibrosis patient for almost 8 years resulted in a mutation rate of 1.3 × 10 −6 changes per site per year [18] . Likewise, sequential Staphylococcus aureus isolates that were taken from the bloodstream of a patient over a period of 3 months revealed a rate of 4.9 × 10 −6 changes per site per year [19] , which was approximately twice the population-based estimate of 2.0–3.3 × 10 −6 for worldwide spreading methicillin-resistant S. aureus lineages [20] , [21] . Mutation rates that are based on phylogenetic comparisons of bacterial populations are usually somewhat lower because of purifying selection that removes a considerable amount of non-synonymous mutations from the population. Accordingly, most changes across the bacterial population affect synonymous sites. Another example for a population-based mutation rate is that from the genomes of the obligate bacterial symbiont Buchnera aphidicola from pea aphids that diversified at a spontaneous mutation rate of 1.4–3.3 × 10 −7 substitutions per site per year over the past 135 years [22] . Somewhat higher mutation rates have been reported for Mycoplasma gallisepticum (0.8–1.2 × 10 −5 ) isolated from house finches and poultry [23] , and for the human pathogens Neisseria gonorrhoeae [24] (4.6 × 10 −5 ) and Campylobacter jejuni [25] (3.2 × 10 −5 ), but those were based on polymorphisms that have predominantly arisen by recombination between isolates rather than by mutation. If we had included recombinant sites, our mutation rate would have been 0.1–3.3 × 10 −2 changes per site per year. Figure 3: Mutation rate versus genome size for bacteria and other biological entities. The estimated H. pylori mutation rate during the acute infection phase was orders of magnitude faster than the mutation rate in other bacteria, comparable to the evolutionary rate of RNA viruses. Data points were taken from references in Supplementary Table 7 . dsDNA, double-stranded DNA; ssDNA, single-stranded DNA. Full size image The mutation burst during the acute H. pylori infection phase was almost as fast as the mutation rate of RNA viruses ( Fig. 3 ) that evolve at a rate of 1.3 × 10 −3 –3.6 × 10 −4 changes per site per year [26] , [27] . We note, however, that mutations in RNA viruses are primarily caused at the level of replication that is not directly comparable to mutations in H. pylori that are likely caused by a combination of replication mistakes and chemical mutagenesis resulting from the immune response. In addition, RNA virus mutation rates have primarily been estimated from phylogenetic comparisons of viral lineages, and were thus likely affected by purifying selection and possibly by population bottlenecks. The significantly high frequency of mutational and recombinant changes in OMP genes of the human re-infection isolates and the J166 output strains suggested selection against bacterial surface structures during the acute infection. Similar to previous observation on J166 output strains from another macaque infection experiment [28] , the hopS ( babA ) gene was either replaced by the closely related OMP gene hopT ( babB ) by intra-chromosomal translocation or contained a frameshift mutation that was caused by an extra CT dinucleotide repeat unit in the 5′ part of the hopS gene ( Supplementary Tables 8–19 ). As was shown previously, either gene conversion or frameshift in the poly(CT) tract functionally inactivates babA , resulting in loss of adherence to the Lewis b blood group antigen on the gastric epithelium [28] . These changes in the H. pylori babA expression in mice and in monkeys typically occurred within the first 4–8 weeks [28] , [29] . In addition, the apparent loss of cag PAI function by frameshift mutations in the cagX and cagY genes ( Supplementary Fig. 2 and Supplementary Tables 14–19 ), as well as by recombination in cagY in mice and in monkeys also happened in this time frame [30] , implying adaptation by mutation and recombination during early stages of the infection. Why did the H. pylori strains, which were isolated from asymptomatic human volunteers, trigger an inflammatory response when re-infecting the same persons? After the original infection was eradicated by antibiotic therapy, the chronic inflammation likely subsided. Following re-infection three months later, resident immune cells in the gastric mucosa such as macrophages and mastocytes detected the re-infecting H. pylori by recognition of general pathogen-associated molecular patterns such as lipopolysaccharide (LPS) and by antibodies. Since several H. pylori OMP genes are variably expressed owing to slipped strand mispairing at homopolymeric nucleotide tracts, this results in growth of clonally related H. pylori with many different sets of expressed OMPs, some of which were likely recognized by antibodies. Subsequently, the immune cells activated the acute inflammatory response by releasing inflammatory mediators such as tumor necrosis factor alpha (TNF-alpha), which then in turn attracted neutrophils (PMNs) to the site of infection. Accordingly, histosections from biopsies taken after the re-infection revealed moderate inflammation, characterized by marked PMN infiltration that extended from the surface into the lamina propria, whereas biopsies taken during the baseline endoscopy showed only mild cellular infiltration, consistent with asymptomatic, chronic H. pylori infection ( Supplementary Fig. 1 ). We cannot rule out the possibility that the patients were originally infected by a mix of strains and not a single strain. However, we cultured a mix of 8–12 colonies for antibiotic sensitivity testing in order to ensure that no resistance had developed to the antibiotics that we planned to use for eradication. All the strains (if more than one) in the stomach at the first endoscopy were sensitive to the six different antibiotics tested (not shown), and the UBTs confirmed eradication. Nevertheless, the detection of numerous CNPs in output strain BM012B, which added up to a total of 173 kb of imported DNA ( Supplementary Table 1 ), suggested (at least transient) co-infection with a different strain, which either was picked up from somebody else sometime between the re-infection and the second endoscopy or was already present in the stomach during the time of the first endoscopy. However, the latter possibility is unlikely because of the two clearly negative UBTs separated by 1 month, which is an excellent proof of cure, at least equal to biopsy and culture. If H. pylori had been present but at undetectably low levels at the time of UBT 1, the chances are very good that the infection would be picked up by the second UBT a few weeks later when more bacteria had re-established themselves. Several factors seem to influence the extent of the acute inflammatory response and thus the level of the mutation burst, including the genetic composition of the bacterial strain such as the alleles of adhesins and the alleles of virulence factors such as cagA or vacA , the number of infecting bacteria, the genetic composition and health of the human (or primate) host and whether the immune system of the host was naive to H. pylori . Consequently, the H. pylori mutation rate during the acute infection phase varied depending on the bacterial strain and host. Although the mutation rates of 8.4 × 10 −4 in the cag PAI-positive strain BM012B and of 6.1 × 10 −4 in the cag PAI-negative strain BM013B from the human volunteers represent the highest estimates so far, the mutation rates of 3.8 × 10 −4 within 1 week to 8.1 × 10 −5 within 1 month in the cag PAI-positive J166 output strains ( Table 2 ) from the immunologically naive macaque were up to one order of magnitude slower. A mutation rate of 4.5 × 10 −5 was derived from 31 SNPs that accumulated in the genome of strain BM012S within 5 months following a naturally occurring transmission of H. pylori strain BM012A between spouses [31] . Extrapolating the accumulation of the 31 SNPs over the 5 months based on the increase in the J166 output strains would result in mutation rates of 5.0 × 10 −4 within 1 week and of 1.6 × 10 −4 within 1 month post infection. All these data contrast the accumulation of just three non-synonymous changes after 3 months of experimental H. pylori infection of another human volunteer [5] . The corresponding mutation rate of 7.5 × 10 −6 , which is similar to that during chronic infection, implies the lack of an inflammatory response in this patient for reasons that are currently unknown, but possibly involved a low number of 10 5 colony-forming units (c.f.u.) in the inoculum [32] in comparison with 10 9 c.f.u. in this re-infection study and to 7.5 × 10 8 c.f.u. in the macaque infection [16] , a cag PAI-negative strain and infection of an immunologically naive host [32] . However, our data show that the inflammatory immune response during the acute infection phase, which is activated by the initial H. pylori infection of the stomach epithelium, triggers a mutation burst in the bacteria ( Fig. 4 ). Since OMP encoding genes appear to be under constant selection by the immune system of the human host, the significantly increased frequency of mutation and recombination events in OMP genes in this (re-) infection study and during naturally occurring H. pylori transmission [31] suggest that changes in immunogenic bacterial surface structures facilitate rapid adaptation of the bacterial pathogen to an individual host. This adaptation process includes evasion of the host’s immune system and will ultimately result in the equilibrium of a chronic infection ( Fig. 4 ). 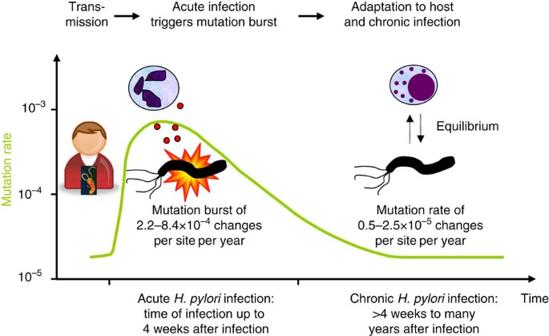Figure 4: Model of the mutation rate over the course of the infection. The initial bacterial infection of the human stomach epithelium activates an acute inflammatory response that triggers a mutation burst in the genome of the bacterial parasite. This mutation burst facilitates rapid adaptation to the individual human host, finally resulting in the equilibrium of a chronic infection. Figure 4: Model of the mutation rate over the course of the infection. The initial bacterial infection of the human stomach epithelium activates an acute inflammatory response that triggers a mutation burst in the genome of the bacterial parasite. This mutation burst facilitates rapid adaptation to the individual human host, finally resulting in the equilibrium of a chronic infection. Full size image Human H. pylori strains and ethics statement The clinical part of this study was performed with written informed consent at the Sir Charles Gairdner Hospital, Nedlands, Western Australia, Australia, under ethics approval 2007-045 by the Human Ethics Committee of this hospital. Antral gastric biopsy specimens were taken from the study participants during gastroendoscopy and cultivated on Pylori agar plates (Biomerieux, Mercy - l’Etoile, France) from which the original ‘input’ isolates, H. pylori strains BM012A and BM013A, were obtained. After single-colony purification, the cultures were split. One part was stored at −80 °C for the subsequent re-infection experiments, and the other part was subjected to DNA isolation for whole-genome sequencing using the Qiagen Blood and Tissue Kit. After the first, ‘baseline’ endoscopy, the human volunteers took eradication therapy with a cocktail of a proton pump inhibitor and three antibiotics (rabeprazole, amoxicillin, clarithromycin and tinidazole), and eradication was confirmed 1 and 2 months later by two consecutive carbon-14 UBTs (PYtest; Kimberly Clark, Utah, USA). According to the procedure guidelines of the Society of nuclear medicine [33] and the manufacturer, reference values of <50 disintegrations per minute (d.p.m.) are considered negative for H. pylori , 50–199 d.p.m. as indeterminate for H. pylori and >200 d.p.m. are interpreted as positive for H. pylori . UBTs were clearly negative for BM012A (0 and 29 d.p.m.) as well as for BM013A (0 and 0 d.p.m.). Three months after the successful H. pylori eradication by antibiotics therapy, the fasting volunteers drank 10 9 c.f.u. of a 2-day-old H. pylori culture suspended in 10 ml of beef broth. Two weeks after swallowing the inoculum, colonization with H. pylori was confirmed by positive UBTs for both BM012A (2,298 d.p.m.) and BM013A (1,108 d.p.m.). Twenty days (strain BM013B) and 44 days (strain BM012B) after the re-infection, endoscopic examination was repeated during which another antral biopsy was taken, from which the two output strains were cultivated. The bacteria were finally eradicated from the study participants. The study was recorded in the Australian Clinical Trial Registry at http://www.anzctr.org.au/trial_view.aspx?ID=82275 . Mucosal biopsies from the first and the second endoscopy were fixed in 10% formalin for histological analysis and processed routinely in the Pathology laboratory by staining with haematoxylin and eosin stain to assess cellular morphology and the presence or absence of bacteria. H. pylori was isolated as single-colony cultures from the output strains, and purified DNA from all four strains was sent to the Pennsylvania State University for whole-genome sequencing. Since no patient information was provided, the study was approved by the ethics board of the Pennsylvania State University as research not involving human participants (IRB no. 35170). Experimental infection of a rhesus macaque All animal procedures were performed at the California National Primate Research Center, which is accredited by the Association for Assessment and Accreditation of Laboratory Animal Care, in compliance with ethical regulations and in accordance with protocols approved by the California National Primate Research Center Research Advisory Committee and by the University of California, Davis, Chancellor’s Animal Use and Care Administrative Advisory Committee. In a previous study, a 4-year-old female rhesus macaque that was confirmed to be free of H. pylori and ‘ Candidatus H. heilmannii’ was inoculated orogastrically with 7.5 × 10 8 c.f.u. of an overnight liquid culture of H. pylori J166 that was resuspended in 1.5 ml fresh brucella broth [16] . The monkey was biopsied at 1 week and 1, 2 and 6 months post inoculation under anaesthesia after an overnight fast. DNA was isolated from J166 and from three H. pylori J166 output strains each that were grown from single colonies from antral biopsies recovered at each of the time points using the Qiagen DNeasy Blood and Tissue Kit. 454-Roche Titanium FLX whole-genome sequencing The genomes strains BM012A, BM012B, BM013A, BM013B and J166 were sequenced to >60 × coverage on a 454-Roche Titanium FLX sequencer. Before library preparation, the quality of the genomic DNA samples was assessed using a Bioanalyzer DNA 7500 Chip (Agilent Technologies). Sample quantitation was performed using Invitrogen’s Picogreen assay. Next-generation sequencing library preparation was performed according to manufacturer’s instructions (Roche Applied Science) with the following modification. The samples were sheared on a Covaris S2 to ~700 bp, following the manufacturer’s recommendation. Library quantitation and emulsion PCR were performed according to manufacturer’s instructions (Roche Applied Science). The libraries were sequenced on a GS FLX instrument using GS FLX Titanium chemistry according to manufacturer’s instructions (Roche Applied Science). The sequence reads were assembled in NEWBLER [34] , and genomic gaps were closed by PCR and Sanger sequencing. The genomes were annotated in RAST [35] , followed by manual curation. Illumina whole-genome shotgun sequencing The genomes of the 12 J166 output strains were sequenced on an Illumina MiSeq. Genomic DNA libraries were created on the automated Agilent Bravo NGS platform using the Illumina TruSeq Nano DNA HT Protocol. Samples were quantified using a Picogreen assay on a TBS-380 Mini-Fluorometer. An amount of 200 ng of sample was fragmented on the Covaris S2 in microtubules. Indexed adapters from the TruSeq Nano HT DNA Sample Prep Kit were ligated into the sheared DNA. Ligated products were purified and size selected to ~570 bp with Sample Selection Beads. The ligated and purified samples were then enriched by eight PCR cycles according to the manufacturer’s protocol. An aliquot of the library was run on the Agilent 2100 Bioanalyzer on a DNA 1000 chip. Library fragments averaged 570 bp, consisting of adapters of ~120 bp and inserts of 450 bp. Sample concentrations were quantified using KAPA Library Quantification Kit using Illumina’s Sequencing Library qPCR Quantification Guide. Samples were normalized to 2 nM. DNA was denatured and loaded onto the MiSeq following the protocol for Illumina MiSeq Reagent kit v2 (500 cycle). Sequencing was performed as a 250 × 250 bp paired-end run with overlapping reads to an average 200 × coverage. Paired-end reads were merged using FLASH [36] and subsequently assembled in NEWBLER [34] . Genome analyses The identified nucleotide changes in strains BM012B and BM013B were validated by aligning the individual sequencing reads of strains BM012B and BM013B against the completed reference genome sequences of strains BM012A and BM013A using INGAP [37] and GSMAPPER implemented in NEWBLER [34] . In addition, SNPs (separated from the next sequence difference by >200 bp of identical sequence on both sides [5] ) were validated by PCR and Sanger sequencing. We assumed that SNPs were introduced by mutation, whereas CNPs (separated by <200 bp and flanked by >200 bp of identical sequence on both sides [5] ) were likely the result of recombination. SNPs ( Tables 1 and 2 ; and Supplementary Tables 1, 2, 4, 8–19 ) were used to calculate the mutation rate, whereby variations in the length of homopolymeric nucleotide tracts of ⩾ 10 bp were not included in the analysis. Likewise, the identified nucleotide changes in the 10 J166 output strains were validated by aligning the individual sequencing reads against the completed reference genome sequence of strain J166. The genomic differences ( Fig. 1 and Supplementary Fig. 2 ) were plotted using GenomeViz [38] . For DNA fragments that were presumably introduced by recombination ( Supplementary Tables 1, 3, 5, 8–19 ), we searched for possible intra-chromosomal DNA donor sources using the Artemis Comparison Tool [39] . Only recombinant DNA fragments that lacked a possible source for intra-chromosomal recombination were assumed to have arisen by DNA import from an unrelated strain. The recombinant fragments in strains BM012B and BM013B were used to estimate the DNA import rate ( Supplementary Table 1 ). The Box-and-Whisker plots ( Fig. 2 ) were generated in R [40] based on the number of mutations and the corresponding mutation rates in Table 2 . The band inside the box represents the median, and the bottom and the top of the box represent the first and the third quartiles, respectively. The whiskers, which extend no more than 1.5 times the interquartile range from the box, indicate the range of the data. The R scripts are provided as Supplementary Notes 1 and 2 . The genomes of strains NQ315, NQ352, NQ367 and NQ392 that were isolated from patients with chronic infection [5] were retrieved from GenBank (accession numbers CADE00000000 , CADG00000000 , CADL00000000 and CADI00000000 ), the sequences of the genes involved in mutation and recombination repair ( Supplementary Table 6 ) were extracted using BLAST searches. How to cite this article : Linz, B. et al . A mutation burst during the acute phase of Helicobacter pylori infection in humans and rhesus macaques. Nat. Commun. 5:4165 doi: 10.1038/ncomms5165 (2014). Accession codes: The complete genome sequences have been deposited in Genbank under the accession numbers CP006888 (BM012A), CP007605 (BM012B), CP007604 (BM013A), CP007606 (BM013B) and CP007603 (J166). The Whole Genome Shotgun projects of the J166 output strains have been deposited at Genbank under the accession numbers JMGN00000000 (J166 output _1wkA), JMGC00000000 (J166 output _1wkB), JMGD00000000 (J166 output _1wkC), JMGE00000000 (J166 output _1moA), JMGF00000000 (J166 output _1moB), JMGG00000000 (J166 output _1moC), JMGH00000000 (J166 output _2moA), JMGI00000000 J166 output _2moB), JMGJ00000000 (J166 output _2moC), JMGK00000000 (J166 output _6moA), JMGL00000000 (J166 output _6moB), and JMGM00000000 (J166 output _6moC). The versions described in this paper are versions JMGx01000000 .